Osmium isotope evidence for a large Late Triassic impact event Anomalously high platinum group element concentrations have previously been reported for Upper Triassic deep-sea sediments, which are interpreted to be derived from an extraterrestrial impact event. Here we report the osmium (Os) isotope fingerprint of an extraterrestrial impact from Upper Triassic chert successions in Japan. Os isotope data exhibit a marked negative excursion from an initial Os isotope ratio ( 187 Os/ 188 Os i ) of ~0.477 to unradiogenic values of ~0.126 in a platinum group element-enriched claystone layer, indicating the input of meteorite-derived Os into the sediments. The timing of the Os isotope excursion coincides with both elevated Os concentrations and low Re/Os ratios. The magnitude of this negative Os isotope excursion is comparable to those found at Cretaceous–Paleogene boundary sites. These geochemical lines of evidence demonstrate that a large impactor (3.3–7.8 km in diameter) produced a global decrease in seawater 187 Os/ 188 Os ratios in the Late Triassic. The Late Triassic was characterized by several marine and terrestrial biotic turnover events before the end-Triassic mass extinction [1] , [2] . The causes of the end-Triassic mass extinction and Norian-to-Rhaetian biotic turnover events are still the subject of active debate. Catastrophic processes, such as widespread eruption of the Central Atlantic Magmatic Province flood basalts, and extraterrestrial impacts have been proposed to account for the biotic turnover events [1] . Impact ejecta layers have been found in the Norian terrestrial sections [3] , [4] , [5] . A Norian deposit in southwestern Britain contains microspherules and shocked quartz that are typical of impact ejecta layers, and it has been suggested that the Manicouagan impact structure in Canada (100 km diameter; ~215 Ma) may be the source of the spherules [4] , [5] . A Norian impact event has been inferred from a platinum group element (PGE) concentration anomaly, and the presence of Ni-rich magnetite and microspherules, in a claystone layer within middle Norian bedded chert succession in the Sakahogi section, Mino Terrane, central Japan [3] . These claystone samples have high PGE concentrations of up to 11.4 ng g –1 osmium (Os), 41.5 ng g –1 Ir, 46.0 ng g –1 Ru and 20.3 ng g –1 Pt, which are comparable to those found at the Cretaceous–Paleogene (K–Pg) boundary [6] , [7] . Given that PGEs are highly depleted in Earth’s continental crust relative to solar abundances [8] , [9] , these anomalously high PGE abundances may have resulted from a large extraterrestrial impactor, similar to the Chicxulub impact event at the K–Pg boundary [6] , [7] . However, previous studies have proposed that redistribution of PGEs under reducing conditions can account for PGE enrichments in deep-sea sediments [10] , [11] , and it remains unclear as to whether the anomalous PGE concentrations in these middle Norian sediments are of meteoritic origin. Here, to identify the origin of the anomalously high PGE abundances in these Norian sediments from Japan, we conduct an Os isotope study of the sediments [12] , [13] , [14] , [15] . Seawater 187 Os/ 188 Os ratios reflect contributions to the global ocean from riverine ( 187 Os/ 188 Os≈1.4), and hydrothermal and extraterrestrial inputs ( 187 Os/ 188 Os≈0.12–0.13) [15] . Given the distinctive 187 Os/ 188 Os ratios of these inputs and the relatively short residence time of Os in the ocean (several tens of thousand years [16] ), seawater 187 Os/ 188 Os ratios are highly sensitive to changes in these fluxes. For example, Os isotope data have been used to infer that an abrupt decline in seawater 187 Os/ 188 Os ratios occurred during the late Eocene [14] , and at the K–Pg boundary, marking the 65-Ma impact event at Chicxulub in Mexico [13] , [17] . 187 Os/ 188 Os ratios of the Norian bedded chert successions in the Sakahogi section are determined to search for evidence of an extraterrestrial input. To validate our interpretation of the Os isotope record from the Sakahogi section, a complementary Os isotope study is conducted on middle Norian bedded cherts of the Enoura section, located ca . 600 km from the Sakahogi section ( Supplementary Figs S1–S4 ). These bedded cherts are considered to be deep-sea sediments that accumulated in a pelagic, open ocean setting within the paleo-Pacific Ocean (Panthalassa) [18] , [19] , [20] . We reconstruct a high-resolution paleo-seawater Os isotope profile for the middle Norian. The major element geochemical compositions of the bedded chert succession in the Sakahogi section are also obtained to place further constraints on the source of Os in the PGE-enriched layer. Geologic setting and sample collection Chert and claystone samples for Os isotope analysis were collected from the Sakahogi section, Mino Terrane, central Japan, where the PGE geochemistry has previously been investigated [3] ( Supplementary Fig. S2 ). A previous paleomagnetic study of the Sakahogi section suggests that these sediments accumulated in a pelagic, open ocean setting within the low-latitudinal zone of the Panthalassa Ocean [18] , [21] ( Fig. 1 ). The claystone layer with high PGE abundances is 4.4 cm thick. We distinguish lower and upper sedimentary sublayers within the claystone ( Fig. 2 ). The lower sublayer (~8 mm thick) is characterized by high PGE concentrations, and comprises clinochlore-rich chlorite microspherules and Ni-rich magnetite–spinel in a matrix of clay minerals (mainly illite), cryptocrystalline quartz and haematite ( Supplementary Fig. S5 ). The upper sublayer is undisturbed sediments whose constituent minerals are clays (illite) and cryptocrystalline quartz, along with radiolarians, siliceous sponge spicules and conodonts. Biostratigraphic analysis of radiolarians and conodonts dates the deposit to upper middle Norian age ( Fig. 1 ). Given that the constant average sedimentation rate of the middle Norian chert succession is 1.0 mm kyr −1 (ref. 3 ), the deposition of the claystone layer occurred ~1 Myr before the middle/upper Norian boundary (~214 Ma) [22] and the duration of deposition at the studied section (65 cm thick) is estimated to be 0.65 Myr. Previous studies have found no geological or geochemical evidence of hydrothermal activity in the studied bedded chert successions [18] , [19] , [23] . Moreover, the redistribution of PGEs in the studied stratigraphic interval is minor, as there is no evidence of downward diagenetic PGE remobilization from the lower sublayer claystone ( Supplementary Fig. S6 ). 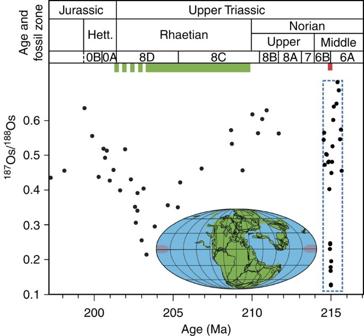Figure 1: Late Triassic Os isotope record in the Panthalassa Ocean. A gradual decrease in187Os/188Os ratios during the Rhaetian (see insert for continental configuration) is considered to have been closely linked with the Central Atlantic Magmatic Province (CAMP) volcanic event (green shaded area)44, whereas the abrupt decrease of187Os/188Os ratios in the middle Norian is synchronous with the ~215 Ma Manicouagan impact event (red bar)3. The blue dashed box outlines the Os isotope data obtained in this study (Fig. 4). The grey circles represent Os isotope data reported by Kurodaet al.44The geologic time scale was taken from Ogg22. The red shaded area on the paleogeographic map shows the estimated depositional site of the bedded chert within the Mino Terrane18. Fossil (radiolarian) zones 6A through 0B are from Onoueet al.3 Figure 1: Late Triassic Os isotope record in the Panthalassa Ocean. A gradual decrease in 187 Os/ 188 Os ratios during the Rhaetian (see insert for continental configuration) is considered to have been closely linked with the Central Atlantic Magmatic Province (CAMP) volcanic event (green shaded area) [44] , whereas the abrupt decrease of 187 Os/ 188 Os ratios in the middle Norian is synchronous with the ~215 Ma Manicouagan impact event (red bar) [3] . The blue dashed box outlines the Os isotope data obtained in this study ( Fig. 4 ). The grey circles represent Os isotope data reported by Kuroda et al . [44] The geologic time scale was taken from Ogg [22] . The red shaded area on the paleogeographic map shows the estimated depositional site of the bedded chert within the Mino Terrane [18] . Fossil (radiolarian) zones 6A through 0B are from Onoue et al . 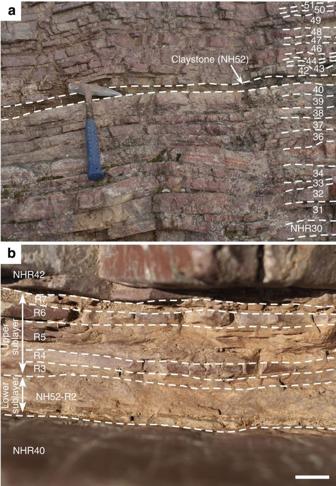Figure 2: Upper Triassic bedded chert of the Sakahogi section. (a) Outcrop view of the claystone bed in the middle Norian bedded chert succession at the Sakahogi section. Numbers NHR30 to 51 refer to individual beds. See bed numbers NHR30 to NHR51 ofFig. 4. (b) Photograph showing detailed occurrence of claystone bed (NH52) at the Sakahogi section. The claystone bed is subdivided into six samples, NH52-R2 to R7 (see text for detail). Note that beds NH52-R4 and R6 contain radiolarians, siliceous sponge spicules and conodonts in a matrix of clay minerals and cryptocrystalline quartz. See bed numbers NH52-R2 to NH52-R7 ofFig. 4. Scale bar, 1 cm. [3] Full size image Figure 2: Upper Triassic bedded chert of the Sakahogi section. ( a ) Outcrop view of the claystone bed in the middle Norian bedded chert succession at the Sakahogi section. Numbers NHR30 to 51 refer to individual beds. See bed numbers NHR30 to NHR51 of Fig. 4 . ( b ) Photograph showing detailed occurrence of claystone bed (NH52) at the Sakahogi section. The claystone bed is subdivided into six samples, NH52-R2 to R7 (see text for detail). Note that beds NH52-R4 and R6 contain radiolarians, siliceous sponge spicules and conodonts in a matrix of clay minerals and cryptocrystalline quartz. See bed numbers NH52-R2 to NH52-R7 of Fig. 4 . Scale bar, 1 cm. Full size image Samples for whole-rock geochemical analysis were collected from 19 chert beds across the claystone layer ( Fig. 2 ). Veins and strongly recrystallized/weathered parts of the chert beds were avoided to minimize the effects of diagenetic or metamorphic overprinting on the sediment geochemistry. We also collected six claystone samples from the lower and upper sublayers. The relatively thick upper sublayer (~3.6 cm) was subdivided into five samples on the basis of colour, lithology, SiO 2 content and biogenic content ( Fig. 2 ). SiO 2 -rich parts of samples NH52-R4 and NH52-R6 contain abundant radiolarians and sponge spicules, and are laterally continuous in the claystone layer ( Fig. 3 and Supplementary Fig. S7 ). 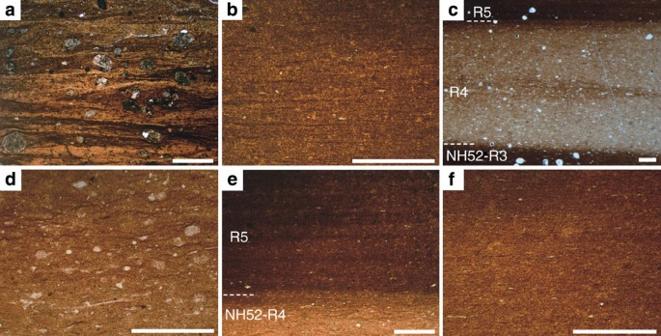Figure 3: Photomicrographs of the claystones from the Sakahogi section. (a) Microspherules from the lower sublayer claystone (NH52-R2). (b) Homogeneous upper claystone (NH52-R3) having no microspherules just above the lower subylayer. (c) Thin intercalation of radiolarian-rich clay (NH52-R4) in the upper sublayer claystone. (d) Abundant radiolarians contained in NH52-R4. (e,f) Crudely laminated clay (NH52-R5) showing no sediment disturbance in the upper sublayer. Scale bars, 500 μm. Plane-polarized light. Figure 3: Photomicrographs of the claystones from the Sakahogi section. ( a ) Microspherules from the lower sublayer claystone (NH52-R2). ( b ) Homogeneous upper claystone (NH52-R3) having no microspherules just above the lower subylayer. ( c ) Thin intercalation of radiolarian-rich clay (NH52-R4) in the upper sublayer claystone. ( d ) Abundant radiolarians contained in NH52-R4. ( e , f ) Crudely laminated clay (NH52-R5) showing no sediment disturbance in the upper sublayer. Scale bars, 500 μm. Plane-polarized light. Full size image To examine whether the Os isotope trends of the Sakahogi section are a global feature, we also studied another middle Norian bedded chert succession from the Enoura section, Chichibu Terrane, southwest Japan ( Supplementary Fig. S8 ). Paleomagnetic analysis of these Triassic bedded cherts, located 600 km from the Sakahogi section, suggests that the depositional setting of these cherts was along the paleo-equator in the Middle Triassic [20] . The Sakahogi cherts accumulated at higher latitudes (16.9°±10.2°N or S) than the Enoura cherts (2.1°±5.2°N or S) during the Middle Triassic, as deduced from paleomagnetic data [20] , [21] , and this indicates that the depositional sites of the two cherts were separated by more than a 1,000 km. At this time, an oceanic plate on which the Enoura Triassic cherts were deposited moved towards the continental margin of East Asia and was accreted during the Middle Jurassic at a lower latitude than the Sakahogi cherts [20] . We analysed nine chert and four claystone samples from the Enoura section ( Supplementary Table S1 ). Re and Os geochemistry Average Re and Os concentrations in the chert samples from the Sakahogi section are 10.5 and 5.4 pg g –1 , respectively, which are much lower than those of the claystone samples ( Supplementary Table S2 ). Os concentrations in the lower sublayer of the claystone (NH52-R2) are as high as 3.0–3.1 ng g –1 and gradually decrease upwards through the upper sublayer (NH52-R3 to NH52-R7) from 0.20 to 0.07 ng g –1 . The lower sublayer is distinctly enriched in Os relative to surrounding sediments, and our results are consistent with those reported by Onoue et al . [3] The lower sublayer of the claystone is characterized by the highest Re concentration (~0.11 ng g –1 ) and lowest Re/Os ratio (~0.03) of the analysed samples ( Fig. 4 ). Re/Os ratios of the chert samples range from 1.00 to 4.19, and are higher than those of the claystone samples. Changes in Re and Os concentrations of the Enoura chert and claystone samples are similar to those of the Sakahogi section, despite the lower sample resolution in the Enoura section ( Supplementary Fig. S8 ). The spherule-rich lower part of the claystone in the Enoura section is also characterized by the highest Os concentrations (~1.2 ng g –1 ) and lowest Re/Os ratios (~0.10) of the studied section ( Supplementary Table S1 ). 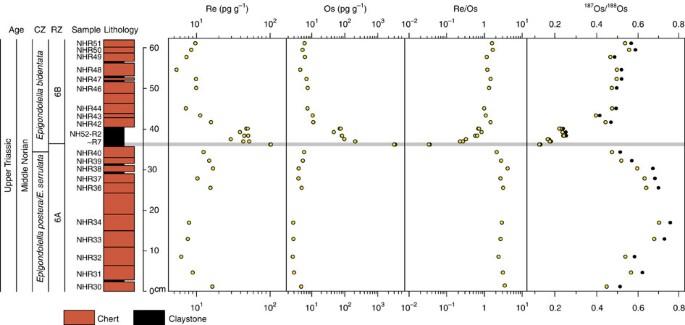Figure 4: Stratigraphic Os isotope profile. Stratigraphic profiles of Re and Os concentrations, Re/Os ratios and Os isotope ratios in bedded cherts of the Sakahogi section. Yellow and black dots in the Os isotope profile represent age-corrected (187Os/188Osi;i=215 Ma) and measured isotope ratios, respectively. The grey shaded line highlights the stratigraphic position of the lower sublayer claystone. Conodont (CZ) and radiolarian (RZ) zones are from Onoueet al.3 Figure 4: Stratigraphic Os isotope profile. Stratigraphic profiles of Re and Os concentrations, Re/Os ratios and Os isotope ratios in bedded cherts of the Sakahogi section. Yellow and black dots in the Os isotope profile represent age-corrected ( 187 Os/ 188 Os i ; i =215 Ma) and measured isotope ratios, respectively. The grey shaded line highlights the stratigraphic position of the lower sublayer claystone. Conodont (CZ) and radiolarian (RZ) zones are from Onoue et al . [3] Full size image Initial Os isotope ratios of the chert samples ( 187 Os/ 188 Os i =0.400–0.704) from the Sakahogi section are relatively homogeneous and higher than those of the claystones. 187 Os/ 188 Os i ratios decline abruptly from 0.477 to 0.126 in the lower sublayer of the claystone ( Fig. 4 ). This marked negative shift in 187 Os/ 188 Os i ratios was confirmed by duplicate analyses ( Supplementary Table S2 ). In the upper sublayer, 187 Os/ 188 Os i ratios gradually increase from 0.178 to 0.234 (NH52-R3 to NH52-R7-1, respectively). Chert samples overlying the claystone layer (NHR42 to NHR51) have 187 Os/ 188 Os i ratios that gradually increase from 0.446 to 0.540, which, on average, are similar to those of chert samples below the claystone (NHR30 to NHR40). The same Os isotope shift is also observed from the Enoura section across the claystone layer ( Supplementary Fig. S8 ). Major element geochemistry The major element compositions of the chert and claystone samples of the Sakahogi section are analogous to the previously published data of the sediments from the Inuyama Area [23] , several hundred metres away from the Sakahogi section, except for the lower sublayer of the claystone ( Supplementary Table S3 ). The negative correlations among SiO 2 versus Al 2 O 3 , MgO and Fe 2 O 3 (total iron as Fe 2 O 3 ) concentrations indicate that our samples have been formed by mixing of biogenic silica (radiolarian test) and terrestrial components (aeolian dusts) derived from the continental crust [23] ( Fig. 5 ). A high Al/(Al+Fe+Mn) ratio indicates that the Sakahogi bedded cherts were deposited in a pelagic deep-sea environment without the affection by hydrothermal activity ( Supplementary Fig. S9 ). The lower sublayer claystone (NH52-R2) exhibits higher MgO, TiO 2 , MnO and Fe 2 O 3 (total iron as Fe 2 O 3 ) concentrations than those of other upper claystone samples. 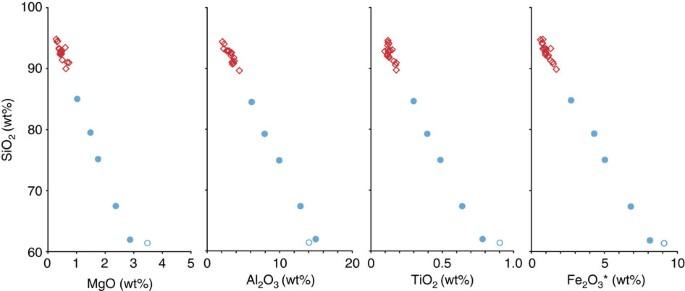Figure 5: Major element compositions of chert and claystone. SiO2versus MgO, Al2O3, TiO2and Fe2O3(total iron as Fe2O3) diagrams of the Sakahogi chert (red open diamonds), and lower (blue open circles) and upper (blue closed circles) claystone samples show negative correlation, indicating mixing of biogenic silica (radiolarian test) and terrestrial components (aeolian dusts) derived from the continental crust23. Figure 5: Major element compositions of chert and claystone. SiO 2 versus MgO, Al 2 O 3 , TiO 2 and Fe 2 O 3 (total iron as Fe 2 O 3 ) diagrams of the Sakahogi chert (red open diamonds), and lower (blue open circles) and upper (blue closed circles) claystone samples show negative correlation, indicating mixing of biogenic silica (radiolarian test) and terrestrial components (aeolian dusts) derived from the continental crust [23] . Full size image Our data from the Sakahogi section reveal the presence of anomalously high Os abundances up to 3.1 × 10 3 pg g –1 within the lower sublayer of the claystone (NH52-R2), which is three orders of magnitude higher than those of the chert samples (~5.4 pg g –1 ). Variations in the Os and other PGE concentrations of the chert and claystone samples are mainly attributable to the different contributions from terrigenous components, apart from the lower sublayer claystone. On the basis of mineralogy and major element chemistry, the claystone samples contain a greater terrigenous component than the chert samples [23] ( Fig. 5 ), suggesting that the higher Os concentrations of the claystone as compared with the chert samples reflects the dominance of terrigenous Os in claystone relative to chert. However, the lower sublayer claystone has extremely high Os concentrations as compared with typical upper continental crust (31 pg g –1 ) [8] , oceanic crust (21–33 pg g –1 ) [24] and other claystone samples from our studied section (NH52-R3, NH52-R5 and NH52-R7). Therefore, the high Os concentrations of the lower sublayer cannot originate from terrigenous input. One possible Os enrichment mechanism is the formation of authigenic ferromanganese minerals in a pelagic deep-water setting [25] , [26] . This mechanism for Os enrichment is, however, inconsistent with the absence of a positive correlation between MnO and Os contents ( Supplementary Tables S2 and S3 ). The lower sublayer samples from the Sakahogi section have unique geochemical signatures, such as anomalously high Os contents (~3.1 × 10 3 pg g –1 ), low Re/Os ratios (~0.03) and unradiogenic 187 Os/ 188 Os i ratios (~0.126), all of which suggest a significant extraterrestrial Os input to the sediments [12] , [14] , [17] . Most meteorites that reach the Earth’s surface (for example, chondrites and irons) have relatively low Re and high Os abundances, and Re/Os≤0.1 (refs 12 , 27 ). In contrast, the continental crust generally has Re/Os>1 (refs 8 , 12 ), as Re is a moderately incompatible element during partial melting of Earth’s mantle. Element abundance ratios of Pt and Ir also support a distinctive PGEs source at the lower sublayer claystone ( Supplementary Fig. S6 ) and indicate a remarkable contribution of meteoritic PGE by an impact event [28] . Moreover, the 187 Os/ 188 Os i ratio of the lower sublayer is similar to that of various chondrite types ( Supplementary Table S4 ). A caveat is that ultramafic rocks with unradiogenic 187 Os/ 188 Os ratio (0.12–0.13) [29] are a highly unlikely source of negative excursion of the lower sublayer claystone, because Os abundances in typical ultramafic rocks (2.6 ng g −1 ) [29] are less than that of the lower sublayer (~3.1 ng g −1 ). Even if the ultramafic rock contains up to 5.2 ng g −1 Os with a 187 Os/ 188 Os ratio of 0.128 (ref. 29 ), a mixing calculation with terrigenous component (31 pg g −1 Os and 187 Os/ 188 Os=1.4) [8] indicates that a ~57% contribution by ultramafic rock is required to explain the high Os concentration of the lower sublayer claystone. On the basis of the detailed field investigation and microscopic observation, we could find no evidence supporting the ultramafic rock contribution, as with the major geochemical compositions of the lower sublayer claystone. The low 187 Os/ 188 Os i ratios in the claystone layer may have been produced by the mixing of ambient seawater Os with meteoritic Os that was vaporized at the time of impact and subsequently dissolved into seawater [14] . A previous petrological study revealed that only the lower sublayer claystone contains abundant spherules and Ni-rich magnetite grains ( Fig. 3 ). Therefore, Os included in the impact-derived particles was added directly into the lower sublayer claystone, not via vaporization and dissolution into seawater. As such, Os isotope data from the lower sublayer claystone were excluded from our reconstruction of the secular variation of ‘seawater’ 187 Os/ 188 Os ratios during the middle Norian impact event. Although our thin-section observations reveal no evidence of bioturbation and reworking (for example, cross stratification, basal or internal scours, reversals or interruptions in grading) in the upper sublayer claystone ( Fig. 3 ), we cannot completely rule out the possibility of contamination from the lower sublayer, induced by the resuspension of bottom currents, especially near the boundary between the lower and upper sublayer claystones (that is, between NH52-R2 and R3). To minimize the possibility of contamination by discrete extraterrestrial particles from the lower sublayer, we excluded the Os isotope values obtained for NH52-R3 when reconstructing the seawater 187 Os/ 188 Os ratio. Except for the lower sublayer and the basal upper sublayer claystones (NH52-R2 and R3), seawater 187 Os/ 188 Os i ratios exhibit a short and marked negative excursion from 0.582 (average 187 Os/ 188 Os i ratios of ten chert samples below the lower sublayer claystone) to 0.222 (average 187 Os/ 188 Os i ratios of four claystone samples of NH52-R4 to R7), which rapidly recovered to 0.446. This abrupt and large change in 187 Os/ 188 Os i ratios provides conclusive evidence for a middle Norian impact event similar to those that occurred in the late Eocene [14] and at the K–Pg boundary [17] . Moreover, the magnitude of this negative 187 Os/ 188 Os i excursion is comparable to those of the late Eocene (0.5 to 0.28) [14] and at the K–Pg boundary (0.4 to 0.157) [17] , and implies that the middle Norian impactor was a large, kilometre-sized object with unradiogenic Os ( 187 Os/ 188 Os i ≈0.12). The size of the impactor can be inferred from the sedimentary Os concentrations and isotope ratios, by making reasonable estimates of the range in the amount of Os released from the impactor into seawater [14] . Estimating the impactor size using such an approach is highly dependent on the assumed nature of the impactor. We consider that the PGEs in the lower sublayer claystone might have originated from a chondrite or iron meteorite, or from one of a small group of PGE-rich achondrites (for example, acapulcoites or ureilites [30] , [31] ). A Howardite–eucrite–diogenite and/or Martian meteorite (shergottite, nakhlite and chassignite) impactor cannot account for the high PGE concentrations in the lower sublayer claystone, as these differentiated achondrites have much lower PGE concentrations (for example, 0.004–3.9 ng g –1 Ir, 0.16–1.4 ng g –1 Pt) [32] , [33] than the lower sublayer claystone (30.0–32.5 ng g –1 Ir, 20.3–23.5 ng g –1 Pt) [3] . Assuming 22 to 100% release of chondrite-derived Os into seawater [6] , [14] , [34] , the impactor is calculated to be 3.3–7.8 km in diameter ( Supplementary Table S4 ). If the impacting object was an iron meteorite that has a higher Os concentration than a chondrite (that is, 35 × 10 3 ng g –1 Os, 187 Os/ 188 Os=0.125, ρ =8 g cm –3 ) [35] , [36] , [37] , and it also released the same amount of Os into seawater (22 to 100%), then the impactor is calculated to be 0.7–1.2 km in diameter. Irrespective of the choice of impactor type, from these calculations it is clear that a kilometre-sized impactor is required to explain the negative Os isotope excursion. The size of the middle Norian impactor, as estimated from the marine Os isotope record obtained in our study, indicates that a large amount of debris and/or climatically active gases (for example, sulphur and carbon dioxide) released from the impact site [6] , [38] , [39] must have affected the physical, chemical and biological environments in the pelagic realm. However, a radiolarian analysis of the Sakahogi [3] and Enoura sections ( Supplementary Table S5 ) provides no evidence for a mass extinction event across the claystone layer. In contrast, significant faunal turnover occurred ~1 Myr after the impact event and 18 radiolarian species became extinct at this level in the bedded chert [3] . It is possible that the impact triggered the extinction of these 18 radiolarian species, although the direct cause of their extinction remains unclear. A recent review of the application of Os isotopes to paleoceanographic studies [40] highlights that our work provides previously undiscovered evidence of a meteoritic Os isotope signature in Triassic deep-sea sediments, which now crop out in an accretionary complex ( Fig. 1 ). It is likely that this impact ejecta layer must also be present in other bedded cherts within other accretionary complexes around the Circum-Pacific. Bedded chert successions, which deposited in the pelagic Pacific Ocean occur in accretionary complexes throughout eastern Russia, Japan, Philippines, New Zealand and western North America. These successions have a wide range of sedimentary ages with a duration of 250 Myr from the Lower Carboniferous to Lower Cretaceous periods. Given that an impact event produced by a chondritic meteorite of 2 km in diameter is detectable using marine Os isotope records [14] , systematic Os isotope studies of these global bedded chert successions should enable the identification of impact events throughout this time. For example, analysis of Os isotope ratios in bedded cherts across the Permian–Triassic boundary [41] would enable testing of the hypothesis that an extraterrestrial impact produced this major biotic extinction event, as has been inferred from the possible discovery of shocked quartz grains and high abundances of Ir in sediments of this age [42] . Re–Os isotope analysis Re and Os concentrations and isotope ratios were determined by isotope dilution–multi-collector–inductively coupled plasma–mass spectrometry (ID–MC–ICP–MS), after Carius tube digestion of samples and sparging introduction of Os into the MC–ICP–MS [43] . PGEs in deep-sea sediments represent subequal inputs by several components, such as aeolian dust, hydrogenetic material and extraterrestrial dust, and the hydrogenetic component can be extracted from bulk samples using this method [44] . We also compared the Re–Os isotope compositions obtained by inverse aqua regia and CrO 3 –H 2 SO 4 digestion for the Sakahogi lower claystone samples and a Triassic chert reference material (JCh-1) issued by the Geological Survey of Japan ( Supplementary Table S6 ). Re–Os data obtained by the two digestion methods are almost identical within analytical uncertainty. Moreover, the variation in the Os isotope records obtained by our Os analytical method for the Upper Triassic bedded cherts of the Inuyama area [44] is positively correlated with marine 87 Sr/ 86 Sr and 187 Os/ 188 Os compositions [45] , [46] , [47] , indicating that Os extracted by our method from the chert samples is dominated by hydrogenous Os. Chert and claystone samples were crushed in an agate mortar and ball mill. Chert samples of ~2.5 g and claystone samples of ~0.5 to ~2.0 g were dissolved and equilibrated with 185 Re and 190 Os spikes in 4 ml of inverse aqua regia, and were heated at 220 °C for 24 h in sealed Carius tubes. Re and Os concentrations and isotope ratios were determined with a Thermo Fisher Scientific Neptune MC–ICP–MS. Total procedural Re and Os blanks were 7.35±0.28 pg ( n =6; average±1 s.d.) and 0.64±0.04 pg ( n =9), respectively, with a 187 Os/ 188 Os ratio of 0.126±0.018 ( n =9) [43] . Initial 187 Os/ 188 Os ratios of the chert and claystone samples were calculated using an age estimated from biostratigraphy and the astronomically tuned geomagnetic polarity time scale (215 Ma; Fig. 1 ), and a 187 Re decay constant of 1.666 × 10 –11 yr −1 (ref. 37 ). Full details of our sample preparation and analytical methods are described in Nozaki et al . [43] Major element analysis Major element (Si, Ti, Al, Fe, Mn, Mg, Ca, Na, K and P) concentrations were determined by X-ray fluorescence spectrometry (XRF). Fused glass beads for XRF analysis were made from a mixture of ~0.4 g of powdered sample and ~4 g of lithium tetraborate flux. All analyses were conducted with a Rigaku Simultix 12 simultaneous wavelength dispersive XRF spectrometer [48] . The accuracy and precision of the XRF analysis were monitored using reference materials of high-Mg basalt (SDSYB) reported by Shimoda et al . [49] , stream sediment (JSd-3) and chert (JCh-1) issued by the Geological Survey of Japan [50] . Estimation of impactor size The diameter of the impacting object d can be calculated by the following equation, with the assumption that 0.22–1.0 to the fraction F of the impact-derived Os dissolved into seawater [6] , [14] , [34] : where ρ impactor (g cm −3 ) and [Os] impactor (ng g −1 ) denote the density and Os concentration of the impactor, respectively. The mass of Os derived from the impactor (mass Os impactor (ng)) is given by following equations [14] : where the seawater Os mass (mass Os sw ) is 1.4 × 10 19 ng (ref. 51 ). 187 Os/ 188 Os postimpact is the 187 Os/ 188 Os i ratio of the upper sublayer claystone (average 187 Os/ 188 Os i ratios of four claystone samples of NH52-R4 to R7; ~0.222), 187 Os/ 188 Os pre-impact is an average 187 Os/ 188 Os i ratio of ten chert samples below claystone layer (NHR30 to NHR40; ~0.582), and 187 Os/ 188 Os impactor is the 187 Os/ 188 Os ratio of the impactor. How to cite this article: Sato, H. et al . Osmium isotope evidence for a large Late Triassic impact event. Nat. Commun. 4:2455 doi: 10.1038/ncomms3455 (2013).